Thermally assisted quantum annealing of a 16-qubit problem Efforts to develop useful quantum computers have been blocked primarily by environmental noise. Quantum annealing is a scheme of quantum computation that is predicted to be more robust against noise, because despite the thermal environment mixing the system’s state in the energy basis, the system partially retains coherence in the computational basis, and hence is able to establish well-defined eigenstates. Here we examine the environment’s effect on quantum annealing using 16 qubits of a superconducting quantum processor. For a problem instance with an isolated small-gap anticrossing between the lowest two energy levels, we experimentally demonstrate that, even with annealing times eight orders of magnitude longer than the predicted single-qubit decoherence time, the probabilities of performing a successful computation are similar to those expected for a fully coherent system. Moreover, for the problem studied, we show that quantum annealing can take advantage of a thermal environment to achieve a speedup factor of up to 1,000 over a closed system. Quantum computation [1] is a computational paradigm that harnesses quantum physics to solve problems. Theory has suggested that quantum computation could provide a significant performance advantage over classical computation. However, efforts to develop useful quantum computers have been blocked primarily due to environmental noise. Adiabatic quantum computation (AQC) [2] , [3] is a scheme of quantum computation that is theoretically predicted to be more robust against noise [4] , [5] , [6] , [7] , [8] , [9] , [10] , [11] , [12] . In AQC, a physical quantum system is initially prepared in its known lowest-energy configuration, or ground state. The computation involves gradually deforming the system’s energy function, or Hamiltonian, in such a way that the system remains in the ground state throughout the evolution with high probability, and the ground state of the final Hamiltonian provides the solution to the problem to be solved. Quantum annealing (QA) [13] , [14] , [15] , [16] is a very similar, but more practical, scheme of quantum computation that is different from AQC in two aspects: the evolution is not required to be adiabatic, that is, the system may leave the ground state due to thermal or non-adiabatic transitions; and the final Hamiltonian is restricted to be diagonal in the computation basis, with a ground state representing the solution to a hard optimization problem. Such optimization problems are integral to a wide range of applications from anthropology [17] to zoology [18] . QA has been experimentally demonstrated in non-programmable bulk solid state systems [19] , [20] and also using 3-qubit nuclear magnetic resonance [21] . Recently, we have designed, fabricated and tested a programmable superconducting QA processor [22] , [23] . Here we report the first experimental exploration of the effect of thermal noise on QA. We explored this using a 16-qubit subset of the processor used in Johnson et al . [23] Closed-system dynamics Our processor implements the Hamiltonian where s≡ t / t f ∈ [0, 1], t is time, t f is the anneal time, are Pauli matrices for the i th qubit, and Δ i ( s ) and Ε ( s ) are time-dependent energy scales. At t =0, Δ i (0)>> Ε (0)≈0, and the ground state is a superposition of all computation basis states, that is, all eigenfunctions of operators. At t = t f , Ε (1)>>Δ i (1)≈0, and H ( s ) is dominated by the Ising Hamiltonian , characterized by dimensionless local biases h i and pairwise couplings J ij . The ground state of H (1) thus represents the global minimum of . Finding this global minimum is known to be an NP-hard (nondeterministic polynomial time hard) optimization problem [24] . An important feature of optimization problems is that, although it may be challenging to find a global minimum, it is easy to select the minimum from a set of candidate solutions, for example, provided by a probabilistic algorithm such as QA. If one is able to find a global minimum with probability P GM >0 in one trial taking time t f , the probability P total of observing a global minimum at least once in k -independent trials, and the total time required t total , is given by For a noise-free (closed) system, P GM would depend on the minimum energy gap, g min , between the ground and first excited states, encountered at some point s = s * known as an anticrossing (illustrated in Fig. 1 ). 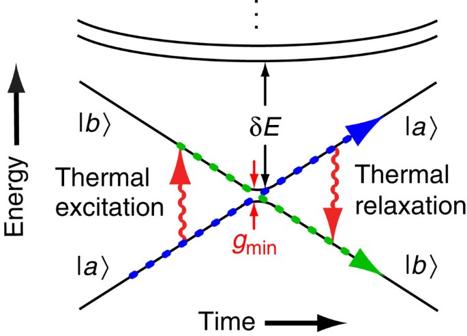Figure 1: Illustration of thermal noise effects near an anticrossing. An avoided crossing (anticrossing) of two lowest-energy eigenstates,and, with a small minimum energy gap,gmin, separated from other eigenstates by energy δE. Passing through the anticrossing very quickly swaps the probabilities of the ground and first excited states (blue and green dotted arrows), leaving the probabilities ofandunchanged. Thus, for a closed-system starting in, the final ground-state probability,Pb, would be vanishingly small. However, with an environment atT>0, thermal transitions can excite the system beforehand and relax it afterward (red arrows), the net effect of which is to increasePb(green arrow). Single-qubit tunnelling amplitudes are significantly larger before the anticrossing (seeFig. 2b), making thermal excitations earlier in the annealing process much more likely than relaxation later. IfT≳δE/kB, higher excited states would also be occupied, reducingPb; so a peak inPbis expected atT=Tpeak∼δE/kB. Using a two-state approximation, one can write [25] , [26] , [9] : Figure 1: Illustration of thermal noise effects near an anticrossing. An avoided crossing (anticrossing) of two lowest-energy eigenstates, and , with a small minimum energy gap, g min , separated from other eigenstates by energy δ E . Passing through the anticrossing very quickly swaps the probabilities of the ground and first excited states (blue and green dotted arrows), leaving the probabilities of and unchanged. Thus, for a closed-system starting in , the final ground-state probability, P b , would be vanishingly small. However, with an environment at T >0, thermal transitions can excite the system beforehand and relax it afterward (red arrows), the net effect of which is to increase P b (green arrow). Single-qubit tunnelling amplitudes are significantly larger before the anticrossing (see Fig. 2b ), making thermal excitations earlier in the annealing process much more likely than relaxation later. If T ≳ δ E / k B , higher excited states would also be occupied, reducing P b ; so a peak in P b is expected at T = T peak ∼ δ E / k B . Full size image where ν =|d( E 1 − E 0 )/d s | s * is the relative slope of the energy levels near s * and t a is the adiabatic timescale, which marks the boundary between adiabatic ( t f >> t a ) and non-adiabatic ( t f << t a ) evolutions. Annealing such a closed system k times, with t f = t total / k , yields the same P total as annealing once with t f = t total . Open-system dynamics In reality, all implementations of quantum algorithms are open systems, and thus subject to relaxation (transitions between energy eigenstates) and dephasing (randomization of relative phases between the eigenstates). In the limit of weak coupling to the environment, dephasing in the energy basis is irrelevant for QA, because only the ground-state probability matters and the relative phases between the energy eigenstates do not carry any information during the computation. Thermal excitation and relaxation, on the other hand, can reduce the instantaneous probability of the ground state by populating the excited states. Nevertheless, in the limit of slow evolution, the ground state will always have the dominant probability, because the excited states are occupied approximately with equilibrium (Boltzmann) probabilities. Unless there are an exponential number of states within the energy k B T ( k B is Boltzmann’s constant) from the ground state, the thermal reduction of the ground-state probability will not significantly affect the performance. This picture changes in the strong coupling limit wherein it may no longer be possible to identify well-defined eigenstates of the system Hamiltonian independent of the environment [27] . It should be noted that, even if the environment is weakly coupled to the system and the equilibrium probability of the ground state is not vanishingly small, the time to reach such a probability is a concern for practical computation. For example, it is conceivable that, due to thermal relaxation, one must wait orders of magnitude longer than a typical closed-system evolution time to reach an acceptable open-system probability. In that case, despite the above argument, the computation cannot be considered robust against the environment. We therefore define robustness against environmental noise as the ability of an open quantum annealing system to yield the correct solution with acceptable probability within a time comparable to the closed-system adiabatic timescale. Experimental results To experimentally investigate the effects of noise on performance, we design an instance of that has an anticrossing with a small g min between an eigenstate , which is a superposition of 256 equal energy (degenerate) local minima of , and an eigenstate , which corresponds to the unique (nondegenerate) global minimum. By studying a small-gap problem, we are addressing what are expected to be the most difficult problems for closed-system AQC (although for an open system, problems with exponentially many low-energy excited states may represent the hardest problems). Moreover, we are interested in exploring evolution during which the minimum gap is passed non-adiabatically, and investigating dependence on annealing time and temperature. To experimentally violate adiabaticity, we require g min / k B <<1 mK. For 16-qubit problems, such small gaps are quite uncommon, and it can be challenging to engineer an instance with sufficiently small g min . Our designed instance is illustrated in Fig. 2a and further described in the Methods section and Supplementary Note 1 . The same type of anticrossing has been argued [28] , [29] to render QA ineffective because of the extremely small g min , though methods have been proposed to eliminate such anticrossings [30] , [31] , [32] . 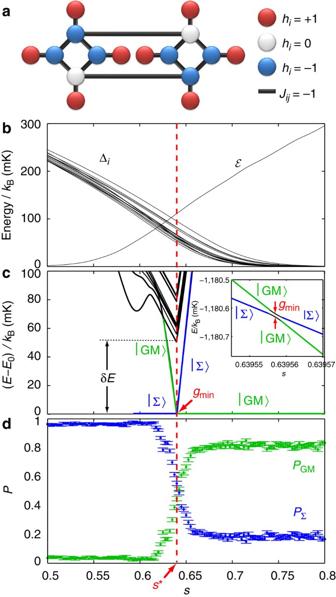Figure 2: The examined problem instance and its energy spectrum. (a) Depiction of the 16-qubit problem instance studied, with corresponding values ofhiandJij. Each circle represents a qubit and each line represents a coupler. The coupling between any two qubits not connected by a line is zero. (b) The energy scales Δi(s) for alliand (s) near the anticrossing. (c) The lowest energy levels of the Hamiltonian, relative to the ground-state energyE0, as a function ofs. States corresponding to the global minimum(green) and the superposition of the 256 local minima(blue) are labelled. The calculated minimum gap isgmin/kB=0.011 mK and δE/kB=50.5 mK. Inset: the lowest two energy levels near the anticrossing. (d) Measured instantaneous probabilities of occupying(green symbols) and(blue symbols) forT=19.9 mK andtf=100 ms. At the anticrossing, both probabilities are ≈0.5. The dashed red line marks the theoretically predicted position of the anticrossing. The error bars depict the s.e.m., assuming each sample is independent. Figure 2: The examined problem instance and its energy spectrum. ( a ) Depiction of the 16-qubit problem instance studied, with corresponding values of h i and J ij . Each circle represents a qubit and each line represents a coupler. The coupling between any two qubits not connected by a line is zero. ( b ) The energy scales Δ i ( s ) for all i and ( s ) near the anticrossing. ( c ) The lowest energy levels of the Hamiltonian, relative to the ground-state energy E 0 , as a function of s . States corresponding to the global minimum (green) and the superposition of the 256 local minima (blue) are labelled. The calculated minimum gap is g min / k B =0.011 mK and δ E / k B =50.5 mK. Inset: the lowest two energy levels near the anticrossing. ( d ) Measured instantaneous probabilities of occupying (green symbols) and (blue symbols) for T =19.9 mK and t f =100 ms. At the anticrossing, both probabilities are ≈0.5. The dashed red line marks the theoretically predicted position of the anticrossing. The error bars depict the s.e.m., assuming each sample is independent. Full size image Of key importance are the energy scales Δ i ( s ) and Ε ( s ) in equation (1), which can be calculated from independently calibrated device parameters (see, for example, Harris et al . [33] and Johansson et al . [34] ). Results for the 16 qubits used in this study are plotted in Fig. 2b . Using these quantities, we calculate the eigenspectrum of H ( s ). Features relevant to this work are found in a narrow region around s ≈0.64, where the anticrossing is expected, as shown in Fig. 2c . The minimum gap, g min / k B =0.011 mK, is more than three orders of magnitude smaller than T ( ≳ 20 mK). The global minimum (green) of is the dominant component of the ground state after the anticrossing, but dominates the first excited state before it. The opposite is true for (blue). Our first objective is to experimentally verify that there is an anticrossing at the predicted position. In the limit of infinitely slow evolution, the instantaneous probability of occupying each eigenstate is approximately given by the Boltzmann distribution. Therefore, the probability P GM ( s ) of occupying should be small before the anticrossing but large after the anticrossing. The opposite should hold for the probability P Σ ( s ) of occupying . The two probabilities should coincide at the anticrossing, where P GM ( s *)= P Σ ( s *)≈0.5. Measuring the instantaneous probabilities P GM ( s ) and P Σ ( s ) would therefore provide information about the approximate position of the anticrossing. We measure the instantaneous probabilities P GM ( s ) and P Σ ( s ) by annealing the system slowly, with t f =100 ms, but interrupting it at s = s d by rapidly moving to s =1 within 20 μs. This rapid evolution takes approximate snapshots of P GM ( s = s d ) and P Σ ( s = s d ). P Σ is determined by summing over the probabilities of observing all 256 local minima of at the end of the evolution. Such a measurement gives a representation of the equilibrium distribution up to some s , beyond which thermal relaxation timescales become exceedingly long (see Supplementary Fig. S5 and Supplementary Note 3 for more details). Figure 2d shows measurements of P GM ( s ) and P Σ ( s ). As expected, P GM ≈1− P Σ ≈0 before the anticrossing. The total probability of states other than the global minimum and the 256 local minima is <0.1%. The two data sets cross near the theoretically predicted s *, where P GM = P Σ ≈0.5. For s > s *, P GM ≈1− P Σ becomes large. As the tunnelling amplitudes Δ i ( s ) are reduced towards the end of annealing, the relaxation between the energy levels becomes slower and slower, and finally the probabilities freeze due to extremely slow relaxation [23] . The ground-state probability at the freeze-out point, therefore, determines the final success probability. As a result, the probabilities saturate for s ≳ 0.66 because of the diminishing relaxation rates between and . (The saturation point and value depend on t f ; see Supplementary Fig. S5 and Supplementary Note 3 .) To examine the impact of noise on QA, we consider the effects of varying T and t f . In the case where t f << t a , passing through the small-gap anticrossing quickly will approximately swap the probabilities of the two crossing states, as depicted in Fig. 1 . For T =0, this would give vanishingly small P GM . Because dominates the excited state just before the anticrossing, increasing T is expected to increase P GM . As T approaches δ E / k B , the energy separation between and , and higher eigenstates, those latter states will be populated, thus reducing P GM . Therefore, a peak in P GM as a function of T is expected at T peak ≲ δ E / k B . 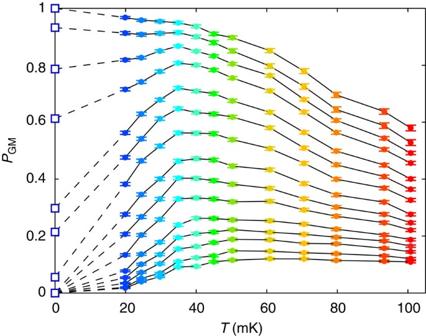Figure 3: Success probability for each anneal time as a function of temperature. Final ground-state probability as a function of temperature for, from top to bottom,tf=500, 200, 100, 50, 20, 10, 5, 2, 1, 0.5, 0.2, 0.1, 0.05, 0.02 and 0.01 ms. The measured temperatures areT=19.9, 24.5, 29.7, 34.9, 40.0, 45.0, 50.3, 60.9, 70.6, 79.7, 93.3 and 100.8 mK. An initial enhancement of the performance is observed with increasingTup toTpeak∼40 mK, in agreement with the theoretical expectation depicted inFig. 1. The blue squares are linear extrapolations of the curves toT=0, subject to 0≤PGM≤1. The error bars depict twice the s.e.m., assuming each sample is independent. Figure 3 shows experimental measurements of the final success probability P GM as a function of T for different t f . All curves, except for those with t f ≥200 ms, show an initial increase with T up to a maximum. For T ≳ 40 mK, the benefits of thermal noise diminish as the system becomes thermally excited to the eigenstates that are at energy δ E / k B ∼ 50 mK above the lowest two states, depicted in Fig. 2c . Figure 3: Success probability for each anneal time as a function of temperature. Final ground-state probability as a function of temperature for, from top to bottom, t f =500, 200, 100, 50, 20, 10, 5, 2, 1, 0.5, 0.2, 0.1, 0.05, 0.02 and 0.01 ms. The measured temperatures are T =19.9, 24.5, 29.7, 34.9, 40.0, 45.0, 50.3, 60.9, 70.6, 79.7, 93.3 and 100.8 mK. An initial enhancement of the performance is observed with increasing T up to T peak ∼ 40 mK, in agreement with the theoretical expectation depicted in Fig. 1 . The blue squares are linear extrapolations of the curves to T =0, subject to 0≤ P GM ≤1. The error bars depict twice the s.e.m., assuming each sample is independent. Full size image It should be emphasized that the enhancement with temperature observed in this experiment is a result of having a small-gap anticrossing separated from all other states by a large energy gap. In more general cases, when several excited states have comparable energy gaps with respect to the ground state with no small-gap anticrossings, increasing T would decrease the probability of success, as observed in Fig. 3 for T >40 mK. The degradation of P GM for high temperatures is instructive, but there is something important to be learned from the low-temperature limit as well. An open system with T =0 has been theoretically predicted to behave similarly to a closed system for such an anticrossing [10] , [35] , [36] , [34] . In this experiment, it was infeasible to reduce T below ∼ 20 mK. Instead, to obtain a crude estimate of P GM at T =0, we extrapolate the curves in Fig. 3 (blue squares). In Fig. 4a , the data shown in Fig. 3 are plotted as a function of t f for different T . We fit (blue dashed line) the formula for closed-system probability, equation (4), to the extrapolated points (blue squares) using t a as the fitting parameter, giving t a =57.2 ms. The fact that the extrapolated points ( T =0) could be fit with equation (4) supports the prediction above. All T> 0 curves fit very poorly to this equation. 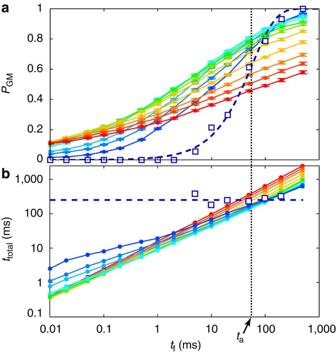Figure 4: Success probability and time to 99% success for each temperature as a function of anneal time. (a) Final ground-state probabilityPGMas a function of annealing time for different temperatures. The error bars depict twice the s.e.m., assuming each sample is independent. (b) Total time required to achievePGM=0.99 by annealing multiple times, as a function of the anneal timetf, computed using equation (3). In both (aandb), temperatures are coloured as inFig. 3, including the extrapolatedT=0 points (blue squares). The dashed blue lines are from fitting the expected closed-system behaviour equation (4) to the extrapolated points, givingta=57.2 ms. ExtrapolatedPGMthat is equal to 0 or 1 yields undefinedttotal. Figure 4: Success probability and time to 99% success for each temperature as a function of anneal time. ( a ) Final ground-state probability P GM as a function of annealing time for different temperatures. The error bars depict twice the s.e.m., assuming each sample is independent. ( b ) Total time required to achieve P GM =0.99 by annealing multiple times, as a function of the anneal time t f , computed using equation (3). In both ( a and b ), temperatures are coloured as in Fig. 3 , including the extrapolated T =0 points (blue squares). The dashed blue lines are from fitting the expected closed-system behaviour equation (4) to the extrapolated points, giving t a =57.2 ms. Extrapolated P GM that is equal to 0 or 1 yields undefined t total . Full size image Despite the influence of thermal noise, it can be seen in Fig. 4a that 0.45 ≲ P GM ≲ 0.8 at t f = t a for all T >0 studied. These probabilities are comparable to P GM =0.63 expected for the closed system. This is because the timescale to reach equal thermal occupation of two anticrossing states is determined by a relaxation time proportional to g min −2 (refs 9 , 10 ), similar to t a in equation (4). It is important to note that for a single, unbiased qubit near s *, we estimate a decoherence time that is millions of times shorter than t a (see Supplementary Note 2 ). The fact that P GM similar to that of a closed system can be reached in time t a , despite the significantly shorter decoherence time, supports theoretical predictions that QA can be performed in the presence of small environmental noise [4] , [5] , [6] , [7] , [8] , [9] , [10] , [11] , [12] . We can also extract the value of g min for this instance based on the value of t a found from the fitting above. In equation (4), ν is only weakly dependent on Hamiltonian parameters, whereas g min is exponentially sensitive [37] . We therefore use the value of ν / k B ≈5.3 K, obtained from the computed spectrum in Fig. 2c , to calculate g min based on the above t a . The result, g min / k B =0.021 mK, is about twice as large as that predicted in Fig. 2c . This is within the expected uncertainty, considering the exponential sensitivity of g min (see Supplementary Note 1 ). Given the values of P GM in Fig. 4a , one can also compare the relative performance of repeated annealing of the QA processor to that of an ideal closed system. Figure 4b shows the total time t total required to achieve P total =0.99 by repeated annealings, as a function of t f , calculated using equation (3). This calculation ignores the overhead for processor preparation and readout, which do not reflect underlying physics. As noted earlier, for the closed system (blue squares and dashed line), t total is independent of t f . For T> 0, t total decreases with decreasing t f , and can be almost three orders of magnitude smaller than that expected for the closed system with t f =0.01 ms. Clearly, in the case of a small-gap anticrossing, such as the one studied here, annealing an open system fast multiple times can have a significant performance advantage over annealing slowly once or annealing a closed system, as predicted [11] . Such an efficiency enhancement due to coupling to the environment has been predicted to have an important role in nature, for example, in photosynthetic quantum energy transfer [38] . In summary, we have found experimental evidence that for a 16-qubit instance with an avoided crossing having an extremely small gap in energy, QA can be robust against thermal noise, well beyond the decoherence time, in line with theoretical predictions. Using a QA processor comprising superconducting flux qubits, we show that the presence of a small amount of thermal noise does not hinder QA in the studied example, and can, in fact, significantly enhance its performance. The thermal enhancement of the performance is restricted to instances with a small-gap anticrossing well separated from other excited states. For general problems with many energy levels thermally occupied during the evolution, increasing T is expected to decrease the final success probability because energy levels within k B T of the ground state may become thermally occupied during the annealing. However, unless the number of these nearby levels increases exponentially with the number of problem variables, the corresponding reduction in ground-state probability can be compensated by repeating the annealing a number of times. These results suggest that QA offers a practical and promising way to perform quantum optimization. The processor The devices studied in this experiment are from a QA processor made of 128 superconducting flux qubits, all controlled by on-chip Single Flux Quantum superconducting digital circuitry as well as filtered analog signal input lines. The qubits are briefly discussed in this section and in detail in Harris et al . [33] The on-chip control circuitry is described in detail in Johnson et al . [39] The qubits are numbered 0–127 starting from the top-left corner of the chip, and the 16-qubit subset used in this experiment is depicted in Supplementary Fig. S2 . Supplementary Fig. S2b represents the qubits as line segments, intersecting at couplers, reflecting the qubit’s physical layout as long, thin radio frequency Superconducting Quantum Interference Device (rf-SQUID) loops. Some of these qubits have been used in previously published experiments. For example, qubit 48 was used in a single-qubit experiment [40] , qubits 48–55 were used in two-qubit experiments [41] , as well as the 8-qubit experiments discussed in Harris et al . [22] and Johnson et al . [23] The annealing procedure we use here is the same as that described in Harris et al . [22] The rf-SQUID flux qubit The qubits used in this experiment are superconducting compound Josephson junction rf-SQUID flux qubits described in detail in Harris et al . [33] A simplified version of the qubit is illustrated in Supplementary Fig. S3 . It has two superconducting loops and therefore two flux degrees of freedom Φ 1 and Φ 2 , subject to external flux biases Φ 1 x and Φ 2 x , respectively. At Φ 1 x ≈Φ 0 /2, the rf-SQUID has two bistable states with persistent current flowing clockwise or counterclockwise through the large loop. These two states form the qubit’s logical ‘0’ and ‘1’ states. The value of the persistent current ( I p ) and the tunnelling amplitude (Δ i ) between the two bistable states are controlled by Φ 2 x . The energy bias between the two states is controlled by Φ 1 x . Supplementary Fig. S4 plots the measured values of I p and Δ i as a function of s for all 16 qubits. Measurement details are provided in Harris et al . [33] The qubits are calibrated to have approximately the same persistent currents, but Δ i is not uniform among the qubits, as is clear from the figure. The overall energy scale E ( s ) in equation (1) is related to the persistent current through , where M 0 is a characteristic mutual inductance determined by the qubit–qubit couplers. Annealing is accomplished by linearly changing Φ 2 x from −0.59Φ 0 at t =0 to −0.65Φ 0 at t = t f . To have a uniform Hamiltonian throughout the evolution, other time-dependent biases are also applied as detailed in Harris et al . [22] The problem instance The instance, shown in Fig. 2a , is designed to have a small energy gap anticrossing, using a phenomenon similar to that presented in Dickson [32] . The eight central qubits in the figure, if unbiased, would have as ground states the all-down and all-up ferromagnetically ordered states. Additional qubits are attached in such a way as to cause 255 more states, close to the all-up state and far from the all-down state, to become degenerate with these states. Then, biases on the central qubits are adjusted to raise the energy of the 256 nearby states, relative to the all-down state, . Repulsion of the 256 degenerate states due to tunnelling between them, away from the end of the evolution, causes the uniform superposition of them, , to be lower in energy than for large enough Δ i ( s ). Because there is a small amount of tunnelling between and , they anticross with a small gap, while being separated from higher energy states by about Δ i ( s *), as shown in Fig. 2c . Additional details can be found in Supplementary Fig. S1 and Supplementary Note 1 . How to cite this article: Dickson, N. G. et al . Thermally assisted quantum annealing of a 16-qubit problem. Nat. Commun. 4:1903 doi: 10.1038/ncomms2920 (2013).